Negative regulation of NF-κB activity by brain-specific TRIpartite Motif protein 9 The TRIpartite Motif (TRIM) family of RING-domain-containing proteins participate in a variety of cellular functions. The β-transducin repeat-containing protein (β-TrCP), a component of the Skp–Cullin–F-box-containing (SCF) E3 ubiquitin ligase complex, recognizes the NF-κB inhibitor IκBα and precursor p100 for proteasomal degradation and processing, respectively. β-TrCP thus plays a critical role in both canonical and non-canonical NF-κB activation. Here we report that TRIM9 is a negative regulator of NF-κB activation. Interaction between the phosphorylated degron motif of TRIM9 and the WD40 repeat region of β-TrCP prevented β-TrCP from binding its substrates, stabilizing IκBα and p100 and thereby blocking NF-κB activation. Consequently, expression or depletion of the TRIM9 gene significantly affected NF-κB-induced inflammatory cytokine production. This study not only elucidates a mechanism for TRIM9-mediated regulation of the β-TrCP SCF complex activity but also identifies TRIM9 as a brain-specific negative regulator of the NF-κB pro-inflammatory signalling pathway. The nuclear factor-κB (NF-κB) transcription factor is a critical regulator of immediate responses to pathogens and also plays an important role in regulating cell proliferation and survival [1] , [2] , [3] . Since unchecked regulation of NF-κB is linked to inflammation, cancer, autoimmune diseases and viral infection, both positive and negative regulation of the NF-κB pathway have been the subjects of intense study [4] , [5] , [6] . NF-κB signalling is divided into the canonical and non-canonical pathways [7] , [8] . Most NF-κB-activating stimuli engage distinct cell-surface receptors (for example, toll-like receptors, interleukin-1 (IL-1) receptor and tumour necrosis factor receptor) or cytoplasmic sensors (retinoic acid-inducible gene I (RIG-I)-like receptors and nucleotide-binding oligomerization domain receptors) through a canonical response, which is dependent on the IκB kinase (IKK) complex. This IKK complex contains the catalytic subunits IKKα and IKKβ, and the scaffold protein NF-κB essential modulator (NEMO; also called IKK-γ) [9] . In non-stimulated cells, NF-κB is held in the cytoplasm in its latent form by a family of inhibitory factors, IκB. Upon stimulation, the IKK complex is activated and phosphorylates the two N -terminal serine residues (S32 and S36) of the inhibitory IκBα protein, triggering recognition and ubiquitination by a complex composed of SKP1–CUL1–F-box protein (SCF) and β-transducin repeat-containing protein (β-TrCP). Ubiquitinated IκBα is consequently degraded through the 26S-proteasome pathway [10] , [11] . Degradation of IκB releases the NF-κB p50/p65 complex from its latent form, allowing nuclear translocation to ultimately result in NF-κB-mediated gene expression. The non-canonical NF-κB pathway involves different signalling molecules that depend on NF-κB2 (p100) processing [12] . Genetic studies show that NF-κB-inducing kinase (NIK) and IKKα [13] are critical kinases for phosphorylation of the C -terminal S866 and S870 residues of p100 to generate the binding motif for β-TrCP [14] . Subsequently, p100 undergoes ubiquitination at its C terminus and degradation, which not only generates the p52 subunit, but also leads to the nuclear translocation of NF-κB to turn on a large number of target genes. Therefore, the SCF-β-TrCP complex plays a central role in both the canonical and non-canonical NF-κB activation pathways. β-TrCP belongs to the F-box protein family. It contains seven C -terminal WD40 repeats that recognize substrates, and an N -terminal F-box that recruits SKP1 to form the so-called SCF E3 complex. β-TrCP is a critical regulator of many cellular processes such as cell cycle, proliferation and development [11] . Mammals have two β-TrCP paralogues with indistinguishable biochemical properties: β-TrCP1 (also known as FBXW1, FBW1A and FWD1) and β-TrCP2 (also known as FBXW11, FBW11, FBXW1B, FBX1B and HOS) and herein β-TrCP is used to represent both of them. β-TrCP is known to recognize the consensus degron (DSGX (2+ n ) S) motif and its variants in which the serine residues are phosphorylated by specific kinases. A number of growth controlling factors have been identified as β-TrCP substrates [15] , including IκBα NF-κB inhibitor, p100 NF-κB precursor, FOXO3 tumour suppressor, Cdc25A cell cycle regulator, β-catenin and Mdm2 oncogenes [11] . In addition, a number of viral proteins are reported to directly or indirectly target β-TrCP. These include the rotavirus protein NSP1 (ref. 16 ), human papilloma virus E7 (ref. 17 ), JC virus large T antigen [18] and human immunodeficiency virus-1 (HIV-1) Vpu [19] . Specifically, HIV-1 Vpu accessory protein downregulates the cell-surface expression of host proteins CD4 and BST-2/tetherin, and subsequently induces their proteolysis via a mechanism involving a β-TrCP SCF E3 ubiquitin ligase complex. While the host regulates β-TrCP activity by modulating its expression, localization or substrate abundance [20] , the direct regulatory mechanisms of β-TrCP activity have not been well elucidated. TRIpartite Motif proteins (TRIMs) are an expanding family containing more than 70 members in humans and mice that are characterized by the presence of a conserved RBCC region: a Really Interesting New Gene (RING) domain, one or two B-Box domains and a predicted Coiled-Coil (CC) domain. They have variable domains at their C termini. TRIM family proteins have been shown to be involved in multiple biological processes and are related to some disorders and diseases [21] , [22] . The N -terminal RING domain is thought to be critical for their ubiquitin E3 ligase activity, and the central B-Box is structurally similar to RING, suggesting that it is also involved in ubiquitination, while the CC domain contributes to homo-oligomeric and hetero-oligomeric interactions. Recent studies have shown that several TRIM proteins play important roles in innate and adaptive immunity, ultimately contributing to intracellular antiviral restriction and regulation of type I interferon (IFN) and NF-κB signalling [23] , [24] , [25] . Among the most interesting and well-characterized TRIMs, TRIM5 is a restriction factor of HIV in old world monkeys [26] ; TRIM25 is essential for RIG-I signal transduction [27] ; TRIM56 positively regulates STING-mediated, double-strand DNA-induced IFN production [28] ; TRIM30 negatively regulates TLR-mediated NF-κB activity [29] and NLRP3 inflammasome [30] ; and TRIM27 negatively regulates IKK-mediated NF-κB activation [31] . Thus, TRIM family proteins play either positive or negative roles in infection-induced host immunity. In order to explore the roles of TRIM family proteins in host innate immune regulation, we screened 62 different TRIM proteins for their activity in the NF-κB signalling pathway and identified TRIM9 as a potent negative regulator of NF-κB activation. TRIM9 is predominantly expressed in the proximal dendrites of neurons in the cerebral cortex and hippocampus, and the Purkinje cells of the cerebellum. Its expression is severely reduced in the affected brain areas in Parkinson’s disease and dementia patients [32] , [33] . Consistent with its potential roles in axonal development, TRIM9 (ref. 6 ) is also highly expressed in the mantle layer of the spinal cord [33] , and its homologues in Caenorhabditis elegans and Drosophila melanogaster have been shown to contribute to neuron development [34] , [35] . In this report, we demonstrate that TRIM9 interacts with the WD repeat region of β-TrCP through its N -terminal degron motif depending on the phosphorylation status. This ultimately stabilizes β-TrCP substrates (IκBα and p100), thereby blocking both canonical and non-canonical NF-κB activation. Our study identifies a novel brain-specific TRIM9-mediated regulatory mechanism of β-TrCP activity that turns off the NF-κB signalling pathway to potentially contribute to brain immune surveillance. TRIM9 efficiently inhibits NF-κB activation We initially investigated the roles of TRIM family proteins in nucleotide-binding oligomerization domain-containing protein 2 (NOD2)-mediated NF-κB activation. To do this, we co-transfected expression vectors for individual TRIM proteins with a NF-κB-luciferase reporter into HEK293-NOD2 cells, followed by stimulation with the NOD2 ligand (L18-MDP) for 24 h. While none of the TRIM proteins robustly stimulated NOD2-mediated NF-κB activation, several of them showed apparent inhibition of NF-κB activation to various degrees ( Fig. 1a ). Specifically, TRIM9 expression showed nearly 10- to 20-fold reduction of NOD2-mediated NF-κB activation ( Fig. 1a ). Further analysis showed that TRIM9 also blocked NF-κB activation induced by various stimulations such as phorbol myristate acetate (PMA)/Ionomycin, IL-1β and tumour necrosis factor (TNF)-α in a dosage-dependent manner ( Fig. 1b ), as well as upon expression of the constitutively active form of intracellular viral RNA receptor RIG-I (RIG-I-2CARD; Fig. 1c ). In contrast, it showed little or no effect on PMA/Ionomycin-induced AP-1 or NF-AT activation, nor on RIG-I-mediated ISRE activation ( Supplementary Fig. 1 ). These results indicate that TRIM9 specifically blocks NF-κB activation from various stimuli. 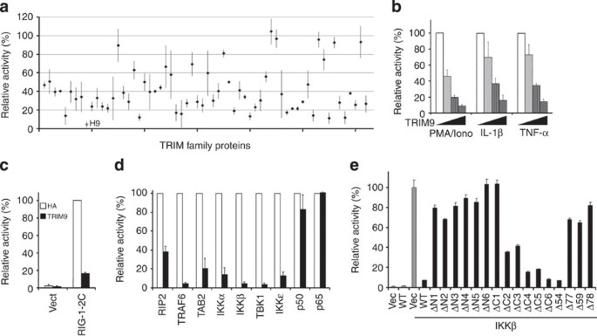Figure 1: TRIM9 expression inhibits NF-κB activation. (a) NOD2-HEK293 cells were transfected with NF-κB and TK-Renilla reporter plasmids together with individual TRIM expression vector for 24 h, stimulated with 10 ng ml−1L18-MDP for 16 h and subjected to dual-luciferase assay. H9: Human TRIM9. (b) At 24 h post transfection with TK-Renilla luciferase transfection control plasmid, NF-κB reporter plasmid and increasing amounts of TRIM9 plasmid (0, 10, 50 and 200 ng), HEK293T cells were stimulated with 50 ng ml−1PMA plus 1 μg ml−1Ionomycin (PMA/Iono), 100 pg ml−1IL-1β or 1 ng ml−1TNF-α overnight and then used for dual-luciferase assay. (c,d) At 24 h post transfection with TK-Renilla luciferase transfection control plasmid, NF-κB reporter plasmid and TRIM9 or vector control, plus plasmids expressing RIG-I 2 CARD (c) or RIP2, TRAF6, TAB2, IKKα, IKKβ, TBK1, IKKɛ, p50, p65 (d). HEK293T cells were used for dual-luciferase assay. White bar: Vector control; black bar: TRIM9. (e,f) At 24 h post transfection with TK-Renilla luciferase transfection control plasmid, NF-κB reporter plasmid and TRIM9 WT or mutants together with IKKβ, HEK293T cells were used for dual-luciferase assay. Results are presented as a percent relative to the activity of cells transfected with vector only. Data (mean and s.e.m.) are representative of at least three independent experiments. Figure 1: TRIM9 expression inhibits NF-κB activation. ( a ) NOD2-HEK293 cells were transfected with NF-κB and TK-Renilla reporter plasmids together with individual TRIM expression vector for 24 h, stimulated with 10 ng ml −1 L18-MDP for 16 h and subjected to dual-luciferase assay. H9: Human TRIM9. ( b ) At 24 h post transfection with TK-Renilla luciferase transfection control plasmid, NF-κB reporter plasmid and increasing amounts of TRIM9 plasmid (0, 10, 50 and 200 ng), HEK293T cells were stimulated with 50 ng ml −1 PMA plus 1 μg ml −1 Ionomycin (PMA/Iono), 100 pg ml −1 IL-1β or 1 ng ml −1 TNF-α overnight and then used for dual-luciferase assay. ( c , d ) At 24 h post transfection with TK-Renilla luciferase transfection control plasmid, NF-κB reporter plasmid and TRIM9 or vector control, plus plasmids expressing RIG-I 2 CARD ( c ) or RIP2, TRAF6, TAB2, IKKα, IKKβ, TBK1, IKKɛ, p50, p65 ( d ). HEK293T cells were used for dual-luciferase assay. White bar: Vector control; black bar: TRIM9. ( e , f ) At 24 h post transfection with TK-Renilla luciferase transfection control plasmid, NF-κB reporter plasmid and TRIM9 WT or mutants together with IKKβ, HEK293T cells were used for dual-luciferase assay. Results are presented as a percent relative to the activity of cells transfected with vector only. Data (mean and s.e.m.) are representative of at least three independent experiments. Full size image Canonical NF-κB signalling converges on the NEMO/IKKα/IKKβ complex that phosphorylates IκBα [4] ; therefore, overexpression of some critical signalling molecules in this pathway strongly activates NF-κB activity. To determine at which step of the NF-κB activation pathway TRIM9 blocks signalling, we co-expressed TRIM9 with several known mediators of canonical NF-κB signalling, including RIP2, TRAF6, TAB2, TBK1, IKKα, IKKβ, IKKɛ, p50 and p65, and then measured the effect of TRIM9 expression on NF-κB activation. This showed that TRIM9 expression effectively blocked NF-κB activation induced by RIP2, TRAF6, TAB2, TBK1, IKKα, IKKβ or IKKɛ; however, it showed nearly no effect on p50- or p65-mediated NF-κB activation ( Fig. 1d ), suggesting that TRIM9 may function upstream of the p65/p50 NF-κB factor, but downstream of the NEMO/IKK complex. TRIM9 N-terminus is required for NF-κB inhibition TRIM9 contains a RING domain at its N terminus, two B-box domains (B-box1 and B-box2) and a CC domain in its central region and a C -terminal subgroup one signature (COS) box, a Fibronectin III (FN3) domain and a PRY-SPRY domain (also known as B30.2) at its C terminus ( Supplementary Fig. 2a ) [32] , [33] . To map which domain(s) of TRIM9 are required for inhibition of NF-κB activation, various TRIM9 mutants were generated and tested for their ability to block IKKβ-mediated NF-κB activation ( Fig. 1e and Supplementary Fig. 2a ). The N -terminal deletion mutants (ΔN1–ΔN6) of TRIM9 lost their ability to block NF-κB activation, whereas most of the C -terminal deletion mutants (ΔC2–ΔC6) of TRIM9, with the exception of the ΔC1 mutant, were able to block NF-κB activation as strongly as TRIM9 wild type (WT; Fig. 1e ). Furthermore, the Δ54, ΔB1 and ΔB2 mutants showed similar levels of NF-κB inhibitory activity to WT ( Fig. 1e ). By contrast, the Δ77 mutant (deletion of 1–77 aa), Δ59 mutant (deletion of 59–77 aa) and Δ78 mutant (deletion of 78–136 aa) lost their ability to block NF-κB activation ( Fig. 1e ). Similar levels of NF-κB inhibition were observed upon stimulation with PMA/Ionomycin, IL-1β or TNF-α, or co-expression with TRAF6, IKKɛ or TBK1 for TRIM9 WT and Δ54 mutant, but not for Δ77, Δ59 and Δ78 mutants ( Supplementary Fig. 2b,c ). Surprisingly, the E3 ligase-dead CA mutant carrying the C30A/C33A mutations at the N -terminal RING domain still significantly inhibited NF-κB activation, suggesting that the TRIM9 E3 ligase activity is not required for the inhibition of NF-κB activity ( Supplementary Fig. 2d ). These indicate that the N -terminal 54–136 aa region of TRIM9 is necessary for its inhibition of NF-κB activation. TRIM9 interacts with β-TrCP Mass spectrometry analysis of the V5-TRIM9 complex identified β-TrCP1 (also called FBW1A) and β-TrCP2 (also called FBW1B, FBW11) as binding partners ( Fig. 2a ). Co-immunoprecipitation (co-IP) with anti-β-TrCP antibody that reacts with both β-TrCP1 and β-TrCP2 showed the specific interaction between TRIM9 and β-TrCP ( Fig. 2b ). Furthermore, endogenous TRIM9 and β-TrCP interaction was readily detected in neuroblastoma SK-N-AS cells, whereas their interactions were reduced upon depletion of TRIM9 expression ( Fig. 2c,d ). Precise inspection revealed that the N -terminal 54–136 aa region of TRIM9 contains the 75 DSGYGS 80 sequence that matches very well with the degron motif (DSGXXS) recognized by β-TrCP where the two serines are phosphorylated ( Fig. 2e ). Specifically, the C -terminal region of β-TrCP containing seven WD40 repeats recognizes the phosphorylated degron motif of IκBα, and results in its degradation, thereby inducing NF-κB activation [11] . Indeed, TRIM9 WT and Δ54 mutant, which efficiently inhibited NF-κB activity, apparently bound β-TrCP, whereas the TRIM9 mutants (Δ59, Δ78 and ΔN1) that were not able to inhibit NF-κB activity did not bind β-TrCP ( Supplementary Fig. 3a ). Furthermore, the TRIM9 SA mutant, in which the serine residues of the putative degron motif were replaced with alanines (S 76 →A and S 80 →A), neither bound to β-TrCP nor inhibited NF-κB activation induced by PMA/Ionomycin, IL-1β or TNF-α ( Fig. 2e–g ). As also seen with p100, the non-canonical NF-κB pathway substrate of β-TrCP whose S866D/S870D mutant loses β-TrCP-binding activity [36] , the S76D/S80D mutant (SD) of TRIM9 showed the lack of β-TrCP-binding activity, thereby lack of inhibition of NF-κB activation ( Supplementary Fig. 4 ). The C -terminal region of β-TrCP containing seven WD40 repeats bound to TRIM9 WT but not the SA mutant, while the truncated WD40 mutants failed to interact with TRIM9 ( Fig. 2h and Supplementary Fig. 3b,c ). Immunofluorescence microscopy showed that as previously reported [37] , both the TRIM9 WT and the SA mutant appeared to be associated with intracellular cytoskeletons through its COS box region, while β-TrCP was diffuse in the cytoplasm ( Fig. 2i ). Upon co-expression, however, TRIM9 WT and β-TrCP were redistributed into punctate compartments, which were not observed upon with SA mutant expression ( Fig. 2i ). These results demonstrate that TRIM9 and β-TrCP interact through the N -terminal degron motif of TRIM9 and the C -terminal WD40 repeats region of β-TrCP. 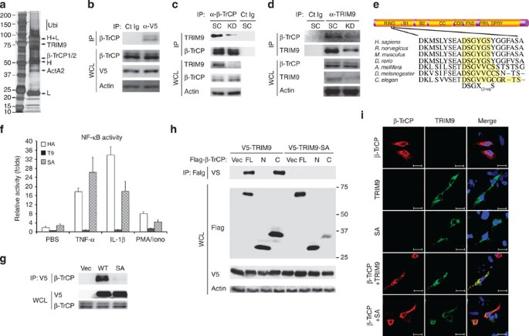Figure 2: TRIM9 interaction with β-TrCP. (a) Anti-V5 immunoprecipitates from 293T-V5-TRIM9 cells were separated by SDS–PAGE and visualized by silver staining. Specific bands were cut and analysed using mass spectrometry. H, IgG heavy chain; L, IgG light chain; ActA2, actin A2. (b) Immunoblot analysis of V5-TRIM9 complexes with anti-β-TRCP. IP, immunoprecipitation; WCL, whole cell lysate. (c,d) SK-N-AS neuroblastoma cells were depleted forTRIM9expression using scramble shRNA or TRIM9-specific shRNA lentivirus and then whole cell lysate (WCL) used for immunoprecipitation (IP) and immunoblotting (IB) with the indicated antibodies. Ct Ig: isotype control immunoglobulin. (e) Diagram of the conserved domains of TRIM9 (upper) and the degron DSGX(2+n)S motif of TRIM9 orthologues (lower). B1, B-Box1; B2, B-Box2; CC, coiled-coil; COS,C-terminal subgroup one signature; FN3, fibronectin type 3; and PRY-SPRY, also known as B30.2. (f) At 24 h post transfection with TK-Renilla luciferase transfection control plasmid, NF-κB reporter plasmid and TRIM9 WT (T9) or SA mutant, HEK293T cells were stimulated with PBS, PMA/Ionomycin, IL-1β or TNF-α overnight and cell lysates were then used for dual-luciferase assay. (g) At 48 h post transfection with Flag-β-TrCP and HA-TRIM9 WT or SA mutant, HEK293T cells were used for IP and IB with the indicated antibodies. (h) At 48 h post transfection with V5-TRIM9 WT or SA mutant together with Flag-β-TrCP full-length (FL),N-terminal region (N) orC-terminal region (C), HEK293T cells were used for IP and IB with the indicated antibodies. (i) Confocal immunofluorescence microscopy of HeLa cells transfected with HA-β-TrCP (red) together with HA-TRIM9 (green) WT or SA mutant. DAPI (blue) was used for nuclear staining. Scale bar=10 μm. The data are representative of three independent experiments. Figure 2: TRIM9 interaction with β-TrCP. ( a ) Anti-V5 immunoprecipitates from 293T-V5-TRIM9 cells were separated by SDS–PAGE and visualized by silver staining. Specific bands were cut and analysed using mass spectrometry. H, IgG heavy chain; L, IgG light chain; ActA2, actin A2. ( b ) Immunoblot analysis of V5-TRIM9 complexes with anti-β-TRCP. IP, immunoprecipitation; WCL, whole cell lysate. ( c , d ) SK-N-AS neuroblastoma cells were depleted for TRIM9 expression using scramble shRNA or TRIM9-specific shRNA lentivirus and then whole cell lysate (WCL) used for immunoprecipitation (IP) and immunoblotting (IB) with the indicated antibodies. Ct Ig: isotype control immunoglobulin. ( e ) Diagram of the conserved domains of TRIM9 (upper) and the degron DSGX (2+ n ) S motif of TRIM9 orthologues (lower). B1, B-Box1; B2, B-Box2; CC, coiled-coil; COS, C -terminal subgroup one signature; FN3, fibronectin type 3; and PRY-SPRY, also known as B30.2. ( f ) At 24 h post transfection with TK-Renilla luciferase transfection control plasmid, NF-κB reporter plasmid and TRIM9 WT (T9) or SA mutant, HEK293T cells were stimulated with PBS, PMA/Ionomycin, IL-1β or TNF-α overnight and cell lysates were then used for dual-luciferase assay. ( g ) At 48 h post transfection with Flag-β-TrCP and HA-TRIM9 WT or SA mutant, HEK293T cells were used for IP and IB with the indicated antibodies. ( h ) At 48 h post transfection with V5-TRIM9 WT or SA mutant together with Flag-β-TrCP full-length (FL), N -terminal region (N) or C -terminal region (C), HEK293T cells were used for IP and IB with the indicated antibodies. ( i ) Confocal immunofluorescence microscopy of HeLa cells transfected with HA-β-TrCP (red) together with HA-TRIM9 (green) WT or SA mutant. DAPI (blue) was used for nuclear staining. Scale bar=10 μm. The data are representative of three independent experiments. Full size image Degron motif phosphorylation is critical for TRIM9 function To test whether serine phosphorylation of the TRIM9 degron motif is required for its interaction with β-TrCP, immunopurified HA-TRIM9 complexes were treated with mock or λ-phosphatase, incubated with lysates containing Flag-β-TrCP and then subjected to immunoblotting with anti-Flag antibody. This showed that treatment of immunopurified TRIM9 with λ-phosphatase drastically abrogated its β-TrCP-binding ability ( Fig. 3a ). Phosphoserine (Sep), the most abundant phosphoamino acid in the eukaryotic phosphoproteome, is not encoded in the genetic code but is synthesized post translationally. Since our attempts to generate the pS 76 pS 80 phospho-specific TRIM9 antibodies failed twice, we utilized the specific cotranslational Sep incorporation system [38] , [39] to study the Ser76 residue of TRIM9. An Escherichia coli strain was genetically engineered to harbour a Sep-accepting transfer RNA (tRNA Sep ), its cognate Sep–tRNA synthetase (SepRS) and an engineered EF-Tu (EF-Sep) of Methanocaldococcus jannaschii , and then transformed with bacterial expression vector containing the N -terminal HA-tagged RING domain (1–160 aa) of TRIM9 WT, the SA mutant and the non-natural Sep-incorporated pS 76 (directed by UAG) mutant ( Fig. 3b ). These HA-TRIM9 proteins were purified from genetically engineered E. coli and used for in vitro pulldown (PD) assay with Flag-β-TrCP. This showed that the pS 76 TRIM9 protein specifically and efficiently bound β-TrCP in vitro , whereas the WT and SA TRIM9 proteins did not bind ( Fig. 3c,d ), suggesting that the serine phosphorylation of the TRIM9 degron motif is necessary for binding the WD40 domain of β-TrCP. 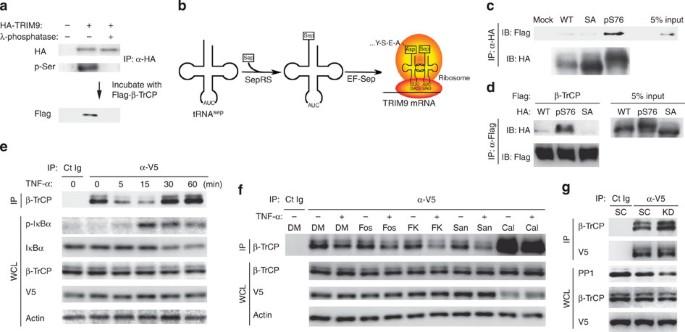Figure 3: TRIM9 interacts with β-TrCP in a phosphorylation-dependent manner. (a) Immunopurified HA-TRIM9 from HEK293T cells was treated with or without λ-phosphatase (500 U) for 30 min at 37 °C. Untreated or λ-phosphatase-treated HA-TRIM9 protein (10%) was used for IB with anti-HA or anti-phospho-serine-specific antibody (p-Ser). The remaining untreated or λ-phosphatase-treated HA-TRIM9 protein was mixed with HEK293T cell lysates containing Flag-β-TrCP for 2 h at 4 °C, washed several times with 1% Tween-PBS washing buffer and subjected to IB with anti-Flag. Data are representative of at least three independent experiments. (b)E. coliBL21ΔSerB strain was engineered with tRNASep(derived fromM. jannaschiitRNACys), SerRS (Sep–tRNA synthetase derived fromM. maripaludisSepRS) and EF-Sep (Engineered phosphoserine-specific EF-Tu). Italicized codon of the TRIM9 mRNA indicates the mutation site (ACG→UAG). Sep: phosphoserine. (c,d)In vitrobinding assay of bacterially purified HA-TRIM9 WT, the Ser76 phosphorylated (pS76) form or the Ser76-to-alanine (SA) mutated form with mammalian Flag-β-TrCP purified from 293T cells. IP with anti-HA and IB with anti-Flag (c) andvise versa(d). (e,f) 293T-TRIM9-V5 cells were stimulated with TNF-α for the indicated times (e) or pretreated with the indicated inhibitors (f), followed by TNF-α stimulation. Cell lysates were used for IP and IB with the indicated antibodies. DM (DMSO control), Fos (Fostriecin, PP2A, 4, 5 inhibitor, 100 μM for 6 h), FK (FK-506, PP2B inhibitor, 100 μM for 6 h), San (Sanguinarine, PP2C inhibitor, 10 mM for 6 h), Cal (Calyculin A, PP1, 2A, 4, 5 inhibitor, 10 nM for 1 h). Ct Ig: isotype control immunoglobulin. (g) At 48 h post infection with lentivirus containing scrambled shRNA (SC) or TRIM9-specific shRNA (KD), 293T cells expressing V5-TRIM9 were used for IP with anti-V5, followed by IB with the indicated antibodies. The data are representative of three independent experiments. Figure 3: TRIM9 interacts with β-TrCP in a phosphorylation-dependent manner. ( a ) Immunopurified HA-TRIM9 from HEK293T cells was treated with or without λ-phosphatase (500 U) for 30 min at 37 °C. Untreated or λ-phosphatase-treated HA-TRIM9 protein (10%) was used for IB with anti-HA or anti-phospho-serine-specific antibody (p-Ser). The remaining untreated or λ-phosphatase-treated HA-TRIM9 protein was mixed with HEK293T cell lysates containing Flag-β-TrCP for 2 h at 4 °C, washed several times with 1% Tween-PBS washing buffer and subjected to IB with anti-Flag. Data are representative of at least three independent experiments. ( b ) E. coli BL21ΔSerB strain was engineered with tRNA Sep (derived from M. jannaschii tRNA Cys ), SerRS (Sep–tRNA synthetase derived from M. maripaludis SepRS) and EF-Sep (Engineered phosphoserine-specific EF-Tu). Italicized codon of the TRIM9 mRNA indicates the mutation site (ACG→UAG). Sep: phosphoserine. ( c , d ) In vitro binding assay of bacterially purified HA-TRIM9 WT, the Ser76 phosphorylated (pS76) form or the Ser76-to-alanine (SA) mutated form with mammalian Flag-β-TrCP purified from 293T cells. IP with anti-HA and IB with anti-Flag ( c ) and vise versa ( d ). ( e , f ) 293T-TRIM9-V5 cells were stimulated with TNF-α for the indicated times ( e ) or pretreated with the indicated inhibitors ( f ), followed by TNF-α stimulation. Cell lysates were used for IP and IB with the indicated antibodies. DM (DMSO control), Fos (Fostriecin, PP2A, 4, 5 inhibitor, 100 μM for 6 h), FK (FK-506, PP2B inhibitor, 100 μM for 6 h), San (Sanguinarine, PP2C inhibitor, 10 mM for 6 h), Cal (Calyculin A, PP1, 2A, 4, 5 inhibitor, 10 nM for 1 h). Ct Ig: isotype control immunoglobulin. ( g ) At 48 h post infection with lentivirus containing scrambled shRNA (SC) or TRIM9-specific shRNA (KD), 293T cells expressing V5-TRIM9 were used for IP with anti-V5, followed by IB with the indicated antibodies. The data are representative of three independent experiments. Full size image Upon TNFα stimulation, the phosphorylated IκBα protein is recognized and ubiquitinated by the SCF-β-TrCP complex and consequently degraded through a proteasome pathway [11] . To investigate the kinetics of TRIM9 and β-TrCP interaction, HEK293T cells stably expressing V5-TRIM9 were stimulated with TNFα, followed by immunoprecipitation for TRIM9 and β-TrCP interaction. While the TRIM9 and β-TrCP interaction was readily detected under no stimulation, it was immediately diminished at 5–15 min following TNFα stimulation and then recovered at 30–60 min following TNFα stimulation ( Fig. 3e ). Conversely, the IκBα phosphorylation was initially undetected without stimulation but robustly increased at 15–30 min after TNFα stimulation ( Fig. 3e ). Ultimately, IκBα degradation was observed at 30–60 min following TNFα stimulation ( Fig. 3e ). Finally, treatment with Calyculin A, an inhibitor for PPase1, 2A and 4/5, considerably increased the TRIM9 and β-TrCP interaction, while other PPase inhibitors, such as FK-506 (PP2B inhibitor), Sanguinarine (PP2C inhibitor) or Fostriecin (PP2A, 4/5 inhibitor), did not do so ( Fig. 3f ). Furthermore, even a marginal depletion of PP1 expression led to an apparent increase in the TRIM9 and β-TrCP interaction ( Fig. 3g ), suggesting that PPase 1 is a primary candidate phosphatase to remove the phosphorylation from the TRIM9 degron motif upon TNF-α stimulation. These data further support that TRIM9 interacts with β-TrCP in a phosphorylation-dependent manner. Effects of TRIM9 on IκBα binding and degradation of β-TrCP To address whether TRIM9 competes with IκBα for β-TrCP binding, TRIM9, β-TrCP and IκBα were expressed in HEK293T cells, followed by an examination of the interaction of β-TrCP with IκBα and TRIM9. This showed that TRIM9 WT, but not the TRIM9 SA mutant, impaired β-TrCP interaction with IκBα in a dosage-dependent manner ( Fig. 4a ). On the contrary, increased expression of IκBα did not significantly block the β-TrCP and TRIM9 interaction ( Supplementary Fig. 5 ). Similarly, when endogenous β-TrCP was immunopurified, its interaction with endogenous phosphorylated IκBα was also diminished in the presence of the TRIM9 WT but not the SA mutant ( Fig. 4b ). Moreover, this reduction was more pronounced upon TNF-α stimulation. Indeed, expression of the TRIM9 WT suppressed the TNF-α-induced ubiquitination of IκBα, whereas expression of the SA mutant did not do so ( Fig. 4c ). 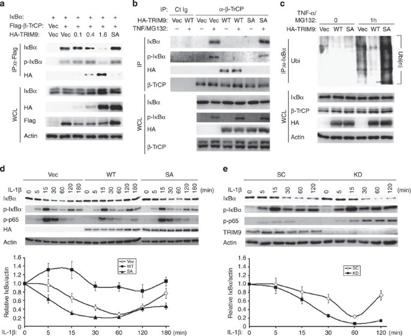Figure 4: TRIM9 competes with IκBα for β-TrCP binding and thereby blocks IκBα degradation. (a) At 48 h post transfection with Flag-β-TrCP and increasing amounts of HA-TRIM9 (μg) or HA-TRIM9 SA mutant, HEK293T cell lysates were used for IP with anti-Flag, followed by IB with anti-IκBα, anti-phospho-specific IκBα or anti-HA antibody. HA-TRIM9 SA mutant was included as a control. (b) HEK293T-HA-TRIM9 or HA-SA mutant cells were treated with TNF-α and 25 μM MG132 for 1 h and cell lysates were used for IP and IB with indicated antibodies. (c) HEK293T cells expressing Vector, HA-TRIM9 WT or the SA mutant were used for IP with anti-IκBα, followed by IB with anti-ubiquitin (Ubi). (d,e) SK-N-AS cells expressing HA-TRIM9 WT or the SA mutant (d) or carrying lentivirus containing scrambled shRNA (SC) orTRIM9-specific shRNA (KD) (e) were stimulated with IL-1β for the indicated times, followed by IB with the indicated antibodies. The IκBα and Actin bands were quantified and the relative IκBα/Actin ratios were used to demonstrate the degradation rate of IκBα (bottom panel). The data are representative of three independent experiments. Figure 4: TRIM9 competes with IκBα for β-TrCP binding and thereby blocks IκBα degradation. ( a ) At 48 h post transfection with Flag-β-TrCP and increasing amounts of HA-TRIM9 (μg) or HA-TRIM9 SA mutant, HEK293T cell lysates were used for IP with anti-Flag, followed by IB with anti-IκBα, anti-phospho-specific IκBα or anti-HA antibody. HA-TRIM9 SA mutant was included as a control. ( b ) HEK293T-HA-TRIM9 or HA-SA mutant cells were treated with TNF-α and 25 μM MG132 for 1 h and cell lysates were used for IP and IB with indicated antibodies. ( c ) HEK293T cells expressing Vector, HA-TRIM9 WT or the SA mutant were used for IP with anti-IκBα, followed by IB with anti-ubiquitin (Ubi). ( d , e ) SK-N-AS cells expressing HA-TRIM9 WT or the SA mutant ( d ) or carrying lentivirus containing scrambled shRNA (SC) or TRIM9 -specific shRNA (KD) ( e ) were stimulated with IL-1β for the indicated times, followed by IB with the indicated antibodies. The IκBα and Actin bands were quantified and the relative IκBα/Actin ratios were used to demonstrate the degradation rate of IκBα (bottom panel). The data are representative of three independent experiments. Full size image To further delineate the mechanism of TRIM9-mediated inhibition of β-TrCP function, we examined IκBα degradation and phosphorylation upon expression of the TRIM9 WT, the SA mutant or genetic depletion of the TRIM9 expression. The IL-1β-induced degradation of IκBα in SK-N-AS neuroblastoma cells was readily suppressed by expression of the TRIM9 WT but not by the SA mutant ( Fig. 4d ). It should be noted that the IL-1β stimulation-induced phosphorylation of IκBα was not significantly changed by expression of either the TRIM9 WT or the SA mutant, suggesting that the IKK activity is not affected by the TRIM9 expression. Conversely, the IL-1β-induced degradation of IκBα was facilitated by the specific short hairpin RNA (shRNA)-mediated depletion of the TRIM9 expression in human SK-N-AS cells ( Fig. 4e ). The S 536 phosphorylation levels of p65, a NF-κB active subunit, were suppressed by TRIM9 expression but enhanced by TRIM9 depletion ( Fig. 4d,e ). Similar results were obtained with human HEK293T cells upon expression of TRIM9 WT or SA mutant ( Supplementary Fig. 6a ) and with human A549 lung epithelial cells upon depletion of the TRIM9 expression ( Supplementary Fig. 6b,c ). These data show that TRIM9 inhibits NF-κB activity by suppressing IκBα degradation. TRIM9 inhibits non-canonical pathways of NF-κB activation As β-TrCP also plays a critical function in non-canonical NF-κB activation by converting the NF-κB precursor p100 to p52 (ref. 14 ), we tested the effect of TRIM9 expression on the master NIK-induced activation of non-canonical NF-κB signalling. In correlation with β-TrCP interaction, TRIM9 WT and the ΔN54 mutant effectively blocked NIK-induced NF-κB activation; however, the SA and ΔN1 mutants failed to do so ( Fig. 5a ). As previously reported [12] , NIK expression induced β-TrCP-mediated processing of p100 to p52 in HEK293T cells; however, TRIM9 expression considerably blocked this process in a β-TrCP-binding-dependent manner ( Fig. 5b,c ). Finally, β-TrCP also bound to p100 in the presence of NIK expression, but this was abrogated by the expression of TRIM9 WT and enhanced by expression of the SA mutant ( Fig. 5c ). Furthermore, upon stimulation of Raji cells with α-CD40 antibody ( Fig. 5d ) or stimulation of A549 cells with LTβ ( Fig. 5e ), overexpression of WT TRIM9, but not the SA mutant, decreased IL-6 production while depletion of TRIM9 expression increased IL-6 production. These results collectively demonstrate that TRIM9 effectively blocks β-TrCP-mediated canonical and non-canonical NF-κB activation. 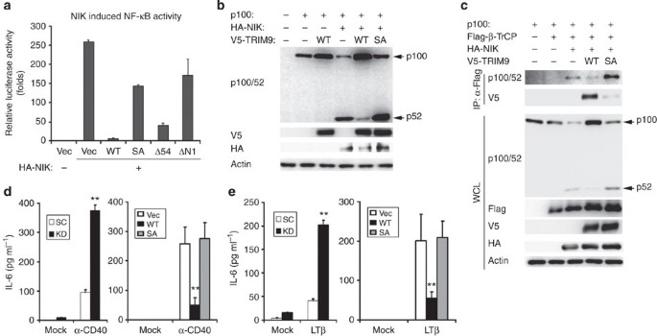Figure 5: TRIM9 inhibits NIK-mediated non-canonical NF-κB processing. (a) At 24 h post transfection with NF-κB reporter plasmid, NIK and HA-TRIM9 WT or its mutants, HEK293T cells were used for dual-luciferase assay. (b,c) At 48 h post transfection with p100, HA-NIK and TRIM9 WT or SA mutant, HEK293T cell lysates were used for IB with the indicated antibodies. (c) At 48 h post transfection with p100, Flag-β-TrCP, HA-NIK, TRIM9 WT or SA mutant, HEK293T cell lysates were used for IP with anti-Flag and IB with anti-p100/52 or anti-TRIM9 antibody. Whole cell lysate (WCL) was used for IB with the indicated antibodies. Arrows indicate the precursor p100 protein and the processed p52 protein. (d,e) Upon depletion ofTRIM9expression (left panel) or expression of TRIM9 WT or SA mutant (right panel), human Raji B cells were treated with α-CD40 (d) and A549 epithelial cells were treated with LTβ (e) for 24 h and their supernatants were subjected to IL-6 ELISA. The mean±s.d. is shown: **P<0.01. The data are representative of three independent experiments. Figure 5: TRIM9 inhibits NIK-mediated non-canonical NF-κB processing. ( a ) At 24 h post transfection with NF-κB reporter plasmid, NIK and HA-TRIM9 WT or its mutants, HEK293T cells were used for dual-luciferase assay. ( b , c ) At 48 h post transfection with p100, HA-NIK and TRIM9 WT or SA mutant, HEK293T cell lysates were used for IB with the indicated antibodies. ( c ) At 48 h post transfection with p100, Flag-β-TrCP, HA-NIK, TRIM9 WT or SA mutant, HEK293T cell lysates were used for IP with anti-Flag and IB with anti-p100/52 or anti-TRIM9 antibody. Whole cell lysate (WCL) was used for IB with the indicated antibodies. Arrows indicate the precursor p100 protein and the processed p52 protein. ( d , e ) Upon depletion of TRIM9 expression (left panel) or expression of TRIM9 WT or SA mutant (right panel), human Raji B cells were treated with α-CD40 ( d ) and A549 epithelial cells were treated with LTβ ( e ) for 24 h and their supernatants were subjected to IL-6 ELISA. The mean±s.d. is shown: ** P <0.01. The data are representative of three independent experiments. Full size image TRIM9 blocks NF-κB-induced inflammatory cytokine production We then tested whether TRIM9 expression affected NF-κB-mediated production of inflammatory cytokine IL-6. HEK293T cells were transfected with TRIM9 or the SA mutant, stimulated with TNF-α, IL-1β or PMA/Ionomycin for 24 h, followed by enzyme-linked immunosorbent assay (ELISA) to detect IL-6 production. This showed that TRIM9 WT but not the SA mutant inhibited stimulation-induced IL-6 production ( Fig. 6a ). Conversely, shRNA-mediated depletion of TRIM9 expression in A549 cells increased IL-6 production upon IL-1β, TNF-α or PMA/Ionomycin stimulation ( Fig. 6b ). Similar results were obtained with SK-N-AS cells upon TRIM9 expression or depletion ( Supplementary Fig. 7 ). 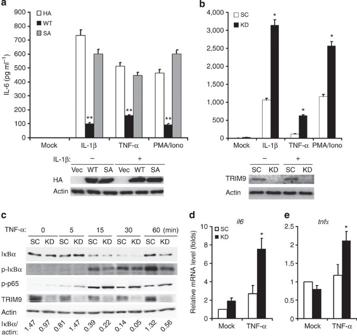Figure 6: TRIM9 inhibits IL-6 inflammatory cytokine production. (a) At 48 h post transfection with vector, TRIM9 WT or SA mutant, HEK293T cells were stimulated with IL-1β, TNF-α or PMA/Iono overnight. The supernatants were then subjected to ELISA to measure IL-6 production. (b) A549 cells carrying lentivirus containing scrambled shRNA (SC) orTRIM9-specific shRNA (KD) were stimulated with IL-1β, TNF-α or PMA/Iono overnight. The supernatants were subjected to ELISA to measure IL-6 production. WCL was used for IB with the indicated antibodies. (c) Primary rat neurons were harvested and infected with scrambled shRNA (SC) orTRIM9-specific shRNA lentivirus (KD), followed by TNF-α stimulation for 2 h. Primary neuron cells were used for IB with the indicated antibody (c) or for real-time RT–PCR to measureil6mRNAs (d) andtnfαmRNAs (e). The IκBα and Actin bands were quantified and the relative IκBα/Actin ratios are presented at the bottom of (c). The mean±s.d. is shown: *P<0.05, **P<0.01. The data are representative of three independent experiments. Figure 6: TRIM9 inhibits IL-6 inflammatory cytokine production. ( a ) At 48 h post transfection with vector, TRIM9 WT or SA mutant, HEK293T cells were stimulated with IL-1β, TNF-α or PMA/Iono overnight. The supernatants were then subjected to ELISA to measure IL-6 production. ( b ) A549 cells carrying lentivirus containing scrambled shRNA (SC) or TRIM9 -specific shRNA (KD) were stimulated with IL-1β, TNF-α or PMA/Iono overnight. The supernatants were subjected to ELISA to measure IL-6 production. WCL was used for IB with the indicated antibodies. ( c ) Primary rat neurons were harvested and infected with scrambled shRNA (SC) or TRIM9 -specific shRNA lentivirus (KD), followed by TNF-α stimulation for 2 h. Primary neuron cells were used for IB with the indicated antibody ( c ) or for real-time RT–PCR to measure il6 mRNAs ( d ) and tnfα mRNAs ( e ). The IκBα and Actin bands were quantified and the relative IκBα/Actin ratios are presented at the bottom of ( c ). The mean±s.d. is shown: * P <0.05, ** P <0.01. The data are representative of three independent experiments. Full size image TRIM9 is predominantly expressed in neurons in the cerebral cortex and hippocampus [33] , and its homologues in C. elegans and D. melanogaster have been shown to contribute to neuron development [34] , [35] . To test whether TRIM9 expression also blocks NF-κB activation in neurons, primary neurons from rat brains were isolated and infected with lentivirus containing scrambled shRNA or TRIM9 -specific shRNA ( Fig. 6c ). The shRNA-mediated depletion of TRIM9 expression in primary rat neural cells led to the reduced accumulation of p-IκBα, the enhanced degradation of IκBα, the augmented S 536 phosphorylation of p65 and the increased expression of il6 , tnfα and neuronal nitric oxide synthase 1 ( nos1 ) mRNAs upon TNF-α stimulation ( Fig. 6c–e and Supplementary Fig. 8 ). These results indicate that TRIM9 expression effectively suppresses the stimulation-induced production of inflammatory cytokines in neurons, which may contribute to brain immune surveillance. Owing to its central role in NF-κB signalling, activity of the β-TrCP SCF complex has to be tightly regulated. So far, expression, localization and substrate abundance have been identified to be the primary means of regulating β-TrCP SCF complex activity. Over 40 proteins have been identified as substrates recognized by the β-TrCP SCF complex [15] ; however, it remains to be determined whether these substrates compete with each other for β-TrCP binding and whether these substrates or other molecules regulate β-TrCP SCF complex E3 enzymatic activity. Here we identify TRIM9 as a negative regulator of β-TrCP SCF complex activity, comprehensively blocking canonical and non-canonical NF-κB activation. Thus, similar to other TRIM family members, TRIM9 restricts host immunity; otherwise, continuous NF-κB-mediated signalling could lead to deleterious effects on the host such as inflammation, cancer, autoimmune diseases and viral infection. TRIM9 is highly expressed in embryonic and adult stages of the brain [32] and its expression is not significantly affected by TNF-α, IL-1β lipopolysaccharide, influenza virus or type I IFN challenge [40] ( Fig. 4e and Supplementary Fig. 6b,c ). Although TRIM9 is recognized as a substrate by β-TrCP, rather than functioning as a substrate, it competes with other substrates for β-TrCP binding, thereby deregulating β-TrCP SCF complex activity. This feature of TRIM9 is similar to that of hnRNP-U [41] and HIV-1 Vpu accessory protein [19] , which are also recognized by β-TrCP through their degron motifs. In fact, Vpu has also been shown to inhibit IκBα degradation in a manner similar to TRIM9 (ref. 42 ). A common feature of TRIM9 and β-TrCP is that their interaction did not lead to a reduction in their protein levels but rather an alteration in the intracellular localization of TRIM9 and β-TrCP: specifically, upon binding, TRIM9 and β-TrCP were redistributed into punctate cytoplasmic compartments. TRIM9 has been shown to be a neuron-specific component of a SNARE (soluble N -ethylmaleimide-sensitive fusion protein-attachment protein receptor) complex associated with synaptic vesicle release control [43] as well as with the cytoskeleton through its COS box region [37] . These associations may ultimately contribute to their intracellular relocalizations in a manner reminiscent of RIG-I, which is also associated with the actin cytoskeleton. It is tempting to speculate that TRIM9-mediated recruitment of the β-TrCP SCF complex to cytoplasmic bodies plays two complementary roles. On one hand, it physically separates the β-TrCP SCF complex from its known substrates such as IκBα and p100 NF-κB inhibitors. On the other hand, movement enables β-TrCP SCF complex to encounter a different set of substrates recruited by TRIM9 for ubiquitination, as HIV-1 Vpu accessory protein does [19] . Further study is necessary to prove or disprove this hypothesis. Phosphorylation of the serine residues of the TRIM9 degron is required for β-TrCP interaction since the dephosphorylation (SA) mutation of TRIM9 impaired its ability to bind β-TrCP. In vitro treatment of phosphatase completely eliminated the interaction between TRIM9 and β-TrCP. These suggest that the phosphorylation and dephosphorylation of the degron motif may be potential regulatory mechanisms for TRIM9 function. Indeed, while the interaction between TRIM9 and β-TrCP was detected under normal conditions, it was rapidly diminished and recovered upon stimulation. It is intriguing that the dissociation of TRIM9 and β-TrCP complex occurred before the IκBα phosphorylation and degradation, suggesting that the dephosphorylation of TRIM9 appears to play an important role in its function as a NF-κB regulator. In fact, Calyculin A (inhibitor of PP1, PP2A, PP4 and PP5) or PPase 1 KD dramatically enhanced the interaction of TRIM9 and β-TrCP. This is correlated with the previous findings [44] , [45] , [46] that PP1 activity is increased after TNFα stimulation, and that depleted expression of PP1α decreases NF-κB activity while increased expression of PP1α augments NF-κB activity upon T-cell receptor engagement. Thus, the phosphorylated TRIM9 may be a substrate for PP1α, which ultimately contributes to the regulation of NF-κB activation. Interestingly, TRIM67, which is also selectively expressed in the cerebellum, shows significant structural and sequence homology to TRIM9 (ref. 47 ): both TRIMs have the same structural organization and exhibit 62% identity and 73% homology. More interestingly, it also carries a degron motif at its N -terminal RING domain and efficiently blocks NF-κB activation upon stimulation with PMA/Ionomycin, IL-1β or TNF-α as we showed with TRIM9 (unpublished results). This suggests that targeting and blocking β-TrCP function in the brain may be a common feature of TRIM9 and TRIM67 as checkpoints for NF-κB activation. TRIM9 expression is decreased in the damaged brains of patients with Parkinson’s disease and Lewy body dementia [32] , [33] . Consistently, NF-κB plays important roles in disorders such as epilepsy, stroke, Parkinson’s disease and Alzheimer’s disease [48] and in inflammation [49] . Indeed, NF-κB activity has been reported to be dramatically increased in Parkinson’s disease patients and Alzheimer disease patients compared with that of age-matched healthy controls [50] , [51] . Furthermore, NF-κB signalling has been implicated in the regulation of neuronal axon initiation, elongation, guidance and branching, and dendrite arbor size and complexity [52] . In fact, the C. elegans TRIM9 homologue (MADD-2) was reported to be involved in axon attraction and branching [34] . Thus, the brain-specific expression of TRIM9, and likely TRIM67, may target the β-TrCP SCF complex to tightly regulate NF-κB activity, contributing to immune balance and neuronal axon growth in the brain. Future functional analysis of TRIM9 may provide potential therapeutic benefits for neurodegenerative diseases. Plasmids TRIM1-TRIM32 and TRIM37 were obtained from Dr Andrea Ballabio (Texas Children’s Hospital) [53] ; TRIM35, 39, 41, 43, 44, 46, 47, 52, 58 and 62 were from Dr Walther Mothes (Yale University) [54] ; and TRIM36, 48, 49, 56 59, 60, 61, 63 and 72 were from Open Biosystems and Invitrogen. The expression plasmids for RIG-I-2CARD and TRIM25 were described previously [27] and TRIM34 was obtained from Dr Paul D. Bieniasz (Howard Hughes Medical Institute) [55] , HA-NIK (Addgene plasmid 27554) was from Dr Shao-Cong Sun (MD Anderson Cancer Center) 12 . β-TrCP and NF-κB2 (p100) were received from Dr Michele Pagano (New York University) [56] . TRIM9 and β-TrCP mutants were generated using a PCR site-directed mutagenesis kit (Stratagene) and subcloned into pCDH vector (System Biosciences) or pEBG vector. Lentivirus-shRNAs against TRIM9 were purchased from OpenBiosystem. The plasmid pRL-TK constitutively expressing Renilla luciferase was purchased from Promega. IKKα, IKKβ, p65, p50 and IκBα were gifted by Dr Ebrahim Zandi (University of Southern California) [57] . Firefly luciferase reporter plasmids under the ISRE (ISG54), NF-AT, AP-1 or NF-κB promoters were purchased from Stratagene. TRAF6, TAB2, IKKɛ, TBK1 and ubiquitin-expressing plasmids were described previously [29] . Cells and reagents HEK293T, A549, SK-N-AS and HeLa cells were purchased from ATCC. HEK293-NOD2 stable cells were purchased from Invivogen. HEK293T, A549 and HeLa cells were maintained in DMEM supplemented with 10% fetal bovine serum (FBS) and 100 U ml −1 penicillin–streptomycin. HEK293-NOD2 cells were maintained with 1 μg ml −1 Blasticidin (Invivogen Inc). SK-N-AS cells were maintained in Eagle’s Minimum Essential Medium (ATCC). Polyclonal TRIM9 antibody (Dilution: 1/20,000) was generated by immunization of rabbits with the TRIM9 N -terminal 1–261 aa purified from E. coli . Antibody sources are: TRIM9 mouse monoclonal antibody (6300-1F12; ABNOVA; Dilution: 1/2,000), β-TrCP rabbit monoclonal antibody (D13F10; Cell Signaling; Dilution: 1/2,000), IκBα mouse monoclonal antibody (L35A5; Cell Signaling; Dilution: 1/2,000), phosphorylated IκBα (5A5; Cell Signaling, Dilution: 1/2,000), NF-κB p65 (93H1; Cell Signaling; Dilution: 1/2,000), IκBα rabbit polyclonal antibody (CalBiochem, Dilution: 1/2,000), p100/p52 mouse monoclonal antibody (9D2; Abcam; Dilution: 1/1,000), HA mouse monoclonal (16B12, Dilution: 1/2,000) and rabbit polyclonal antibodies (Covance, Dilution: 1/2,000), Flag mouse monoclonal (M2; Dilution: 1/5,000) and rabbit polyclonal antibodies (Sigma; Dilution: 1/2,000), V5 mouse antibody (Life Technologies; 2F11F7; Dilution: 1/5,000) and rabbit polyclonal antibodies (Bethyl Laboratories; Dilution: 1/2,000), GST polyclonal antibody (Sigma; Dilution: 1/2,000) and Ubiquitin monoclonal antibody (P4D1; Santa Cruz; Dilution: 1/1,000). IL-1β and TNF-α were purchased from R&D; PMA and Ionomycin were purchased from Sigma; siRNA against PPase 1 was purchased from Santa Cruz Biotechnology, Inc. Construction of TRIM9-expressing and knockdown cells A549 and SK-N-AS cells were seeded into six-well clusters overnight and culture medium was replaced with complete growth medium containing 8 μg ml −1 polybrene (Sigma) and 5 × 10 5 infectious units of lentiviruses containing scrambled shRNA, trim9 -specific shRNAs (target sequence for human: 5′- CGATGCCCTCAACAGAAGAAA -3′; for mouse and rat: 5′- AATGTCTTTCTGTTTAAGTCG -3′) or pCDH lentivirus expressing HA-TRIM9 WT or the SA mutant. At 48 h post infection, cells were trypsinized and seeded into 60-mm dishes with complete growth medium containing 2 μg ml −1 puromycin (Invivogen Inc). Puromycin-resistant cells were maintained in growth medium containing puromycin for a maximum of 15 passages. Reporter assays Cells were transfected with the indicated reporters together with pRL-TK transfection control reporter. At 24 h post transfection, cells were treated as indicated in the figure legends, followed by luciferase assay. For TRIM protein screening, HEK293 NOD2 stable cells were seeded in 48-well plates at 2.5 × 10 4 cells per well. At 16 h post seeding, cells from each well were transfected with a total of 250 ng DNA containing 48 ng firefly luciferase reporter plasmid, 2 ng renilla luciferase reporter plasmid (pRL-TK) and individual TRIM plasmids using Lipofectamine 2000 (Invitrogen). All samples were transfected in triplicate. At 24 h post transfection, cells were stimulated with 100 pg ml −1 L18-MDP (Invivogen) for 16 h and then lysed in passive lysis buffer (Promega), and luciferase activity was measured using the Dual-Luciferase Reporter Assay System (Promega) using a Beckman Coulter DTX880 plate reader. Firefly luciferase values were normalized to renilla luciferase values. Fold increase in the firefly reporter was calculated relative to the vector control in each experiment. In addition, HEK293T cells were transfected with the indicated plasmids combined with NF-κB-Luc, AP-1-Luc, NF-AT-Luc or pISRE-Luc reporter (Stratagene), and pRL-TK (Clontech). At 24 h post transfection, cells were lysed or treated with IL-1β, TNF-α and PMA/Ionomycin for 16 h and then reporter luciferase activity was analysed with the Dual-Luciferase Reporter Assay System (Promega). Immunoprecipitation, GST pulldown and immunoblot analysis For co-IPs, cells were lysed with RIPA minimum lysis buffer (Millipore). After clarification and preclearing, protein amounts were determined using BCA assay. Cell extracts were incubated for 12–16 h with the indicated antibodies, followed by additional incubation with protein A/G beads for 2–4 h. Immune complexes were washed with lysis buffer with 400 mM NaCl and subjected to immunoblot analysis. For endogenous co-IP, antibodies were conjugated to resin using the Co-IP kit (Pierce). For ubiquitination assay, cells were initially lysed with RIPA buffer containing 1% SDS, and cell extracts were diluted with RIPA buffer to 0.1% SDS concentration and then subjected to IP and IB. Full scan image of the western blots are provided in Supplementary Fig. 9 . Confocal microscopy At 24 h post transfection, HeLa cells were fixed with 2% paraformaldehyde solution at room temperature for 20 min, permeabilized and stained with antibodies for confocal microscopy (Nikon Eclipse Ti). Anti-mouse HA (TRIM9), anti-rabbit Flag (β–TrCP) anti-mouse and/or anti-rabbit Alexa Fluor-488, and Alexa Fluor-568 antibodies (Invitrogen) were used. Hoechst dye (Invitrogen) was used to stain nuclei. ELISA For overexpression, HEK293T cells were transfected for 24 h with TRIM9 WT, TRIM9 SA or vector. Cells were then stimulated for 24 h with IL-1β, TNF-α or PMA/Ionomycin. SK-N-AS cells stably expressing TRIM9 WT, SA mutant or vector were stimulated with IL-1β for 24 h. For knockdown assay, SK-N-AS and A549 stable knocked down TRIM9 or control cells were stimulated with IL-1β, TNF-α or PMA/Ionomycin, respectively. Supernatants were collected and their concentration of IL-6 or TNF-α was determined with a human-specific ELISA kit (BD Biosciences), followed by analysis with a Beckman Coulter DTX880 plate reader. Q-PCR Total RNAs were extracted from cultured cells with the RNeasy Mini Kit (Qiagen) according to the manufacturer’s instructions. Oligo(dT) priming and Superscript III reverse transcriptase (Invitrogen) were used for reverse transcription of purified RNA. All gene transcripts were quantified by quantitative PCR with iQ SYBR Green supermix and CFX96 real-time PCR system (Bio-Rad). Primers for nos1 : Forward, 5′- GGCGTCCGTGACTACTGT -3′, Reverse, 5′- ATGAAGGACTCCGTGGC -3′; il6 : Forward, 5′- TCCTACCCCAACTTCCAATGCTC -3′, Reverse, 5′- TTGGATGGTCTTGGTCCTTAGCC -3′; tnfα Forward, 5′- AAATGGGCTCCCTCTCATCAGTTC -3′, Reverse, 5′- TCTGCTTGGTGGTTTGCTACGAC -3′; hprt Forward, 5′- CTCATGGACTGATTATGGACAGGAC -3′, Reverse, 5′- GCAGGTCAGCAAAGAACTTATAGCC -3′. Protein purification and mass spectrometry HEK293T cells stable expressing V5-TRIM9 were collected and lysed with NP40 buffer (50 mM HEPES, pH 7.4, 150 mM NaCl, 1 mM EDTA, 1% (v/v) NP40) supplemented with a complete protease inhibitor cocktail (Roche) and phosphatase inhibitors cocktail 3 (Sigma). Post-centrifuged supernatants were pre-cleared with protein A/G beads at 4 °C for 2 h and mixed with mouse anti-V5 and protein A/G beads for 4 h at 4 °C. Precipitates were washed extensively with lysis buffer and separated by SDS–PAGE. After silver staining, specific protein bands were excised and analysed using ion-trap mass spectrometry at the Harvard Taplin Biological Mass Spectrometry facility, and amino-acid sequences were determined using tandem mass spectrometry and database searches. Unnatural amino-acid protein expression The production of HA-tagged TRIM9 N -terminal (1–160 aa)-His 6 WT, the Ser76 phosphorylated form or the SA mutant was followed as described previously in detail [39] . Briefly, the Ser76 (TCG) codon was replaced by the pSer76 (UAG) amber codon or the SA (CGG) mutation codon by site-directed mutategenesis (Stratagene). The expression clones were transformed into E. coli BL21ΔSerB with pKD-SepRS-EF-Tu. E. coli were grown at 25 °C supplemented with 100 μg ml −1 of Amp, 50 μg ml −1 Kan, 12 μg ml −1 Tet, 2 mM Sep, 5,052 solution and phosphate buffer for autoinduction. After induction, E. coli was harvested, lysed, subjected to Ni 2+ -NTA agarose column purification and anion exchange column purification. Finally, purified proteins were separated through SDS–PAGE and stained with Coomassie brilliant blue. Rat neural cell isolation, culture and transfection Sprague–Dawley rats were raised, bred, and maintained in accordance with protocols approved by the USC Institutional Animal Care and Use Committee until euthanasia for neuron isolation. Rat neural precursor cells were obtained from the brain cortex as described elsewhere [58] . Briefly, telencephalons of E14 rat fetuses were dissected and the tissues were incubated with trypsin-EDTA solution (Gibco) for 10 min at 37 °C and then dissociated mechanically. Neural precursor cells were cultured in passaging medium: DMEM/F12 (Gibco), 0.6% glucose, 10 μg Insulin-Transferrin-Sodium Selenite Supplement (Roche), 1% penicillin/streptomycin, 20 ng ml −1 EGF (Sigma); 5 ng ml −1 FGF-2 (Sigma), 5 μg ml −1 heparin (Sigma) and 2% B27 supplement (Gibco) and grown as neurospheres. Then, neurospheres were digested with Accutase (Life Technologies) and plated on coverslips coated with the poly- L -lysine (Sigma) and laminin (Sigma) in differentiation medium (Neurobasal, 2% B27 supplement from Gibco), allowing them to migrate and differentiate for 7 days. Cells were then maintained in an incubator at 37 °C with a 5% CO 2 atmosphere and 95% humidity. For TRIM9 knockdown, neurospheres were digested with Accutase and cultured in passaging medium containing 8 μg ml −1 polybrene (Sigma) and 5 × 10 5 infectious units of lentiviruses containing scrambled shRNA or rat TRIM9-specific shRNA. After 48 h, differentiation medium was added to allow cells to differentiate for 7 days. Statistics One-way analysis of variance was used for multiple-group comparisons, followed by Bonferroni procedure for comparison of means. Student’s t -test was used for the comparison of two independent groups. For all tests, a P value of less than 0.05 was considered statistically significant. How to cite this article: Shi, M. et al . Negative regulation of NF-κB activity by brain-specific TRIpartite Motif protein 9. Nat. Commun. 5:4820 doi: 10.1038/ncomms5820 (2014).